Ultralight nanofibre-assembled cellular aerogels with superelasticity and multifunctionality Three-dimensional nanofibrous aerogels (NFAs) that are both highly compressible and resilient would have broad technological implications for areas ranging from electrical devices and bioengineering to damping materials; however, creating such NFAs has proven extremely challenging. Here we report a novel strategy to create fibrous, isotropically bonded elastic reconstructed (FIBER) NFAs with a hierarchical cellular structure and superelasticity by combining electrospun nanofibres and the fibrous freeze-shaping technique. Our approach causes the intrinsically lamellar deposited electrospun nanofibres to assemble into elastic bulk aerogels with tunable densities and desirable shapes on a large scale. The resulting FIBER NFAs exhibit densities of >0.12 mg cm −3 , rapid recovery from deformation, efficient energy absorption and multifunctionality in terms of the combination of thermal insulation, sound absorption, emulsion separation and elasticity-responsive electric conduction. The successful synthesis of such fascinating materials may provide new insights into the design and development of multifunctional NFAs for various applications. Ultra-low density materials are attractive for their wide range of applications in the fields of thermal insulation, catalyst supports, tissue engineering, battery electrodes and acoustic, vibration or shock energy damping [1] , [2] , [3] , [4] . The ultralight regime below 10 mg cm −3 currently contains very few materials: silica colloid aerogels (>1 mg cm −3 ), carbon nanotube aerogels (>0.16 mg cm −3 ), graphene monoliths (>0.5 mg cm −3 ), aerographite (>0.18 mg cm −3 ), and metal microlattices (>0.9 mg cm −3 ) (refs 5 , 6 , 7 , 8 , 9 ). All of these ultra-low density materials have cellular architectures, which are synthesized by the assembly of various building blocks, such as colloidal particles, nanotubes, graphene, nanorods and so on. The effective properties of the ultralight cellular materials are defined both by their cell geometry (that is, the spatial configuration of voids and the solid) and the properties of the solid constituents (for example, strength, continuity and so on) [9] , [10] , [11] . In natural structures, it has been demonstrated that introducing a continuous fibrous structure can substantially improve material utilization and the resultant properties [12] , [13] , [14] . For instance, spider webs possess a relative density similar to that of ultralight aerogels but are clearly structurally robust [15] . Inspired by this idea, creating three-dimensional (3D) nanofibrous aerogels (NFAs) with high continuity and an open-cell cellular structure could be another strategy for achieving promising performance for widespread applications. Several cellulosic materials, including bacterial cellulose fibrils, cellulose nanocrystals and lignocellulose, have recently been used as building blocks and assembled into NFAs [16] , [17] , [18] . However, the inherent limits on the diversity of bulk materials, combined with the lack of precise control of the physicochemical and mechanical properties, present major challenges in the synthesis of NFAs that must be addressed before their extensive practical applications. Electrospun nanofibres, which are at the forefront of advanced fibrous materials, combine the robust mechanical strength, low density, fine flexibility, extremely high aspect ratio and ease of scalable synthesis from various materials (polymer, ceramic, metal, carbon and so on) [19] , [20] , [21] . These fibres hold great promise as an exceptional nanoscale building block for constructing macroscopic NFAs. Despite their outstanding potential, the major problem associated with electrospun nanofibres is their anisotropic lamellar deposition character, with the resultant nanofibres usually assembling into close-packed membranes (with thicknesses <100 μm) rather than into bulk aerogels [22] , [23] . Current knowledge on the 3D shaping of electrospun nanofibres suggests that the NFAs should be prepared by stacking layers of nanofibre membranes together or by using specially designed fibre collectors [23] , [24] , [25] . However, the principle of these methods remains the direct deposition of nanofibres; thus, the anisotropic lamellar deposition problem of electrospun fibres has not been solved. Moreover, most of these products are not real 3D-structured aerogels but rather stacks of membranes or fluffy cotton-like nanofibre deposits, which exhibit poor mechanical strength with no elastic resilience [25] , [26] . The challenge, therefore, is to construct homogeneous, continuous and mechanically robust NFAs capable of forming a 3D isotropic cellular architecture, without compromising the functionality of the intrinsic nanofibres. In this work, we present a robust methodology for creating superelastic NFAs with a hierarchical cellular structure that consists of bonded nanofibres, which we call ‘fibrous, isotropically bonded elastic reconstructed’ (FIBER) NFAs. The premise for our design is that the intrinsically lamellar deposited electrospun nanofibres are reconstructed into 3D elastic bulk aerogels with tunable densities and desirable shapes on a large scale. We demonstrate that our FIBER NFAs exhibit the integrated properties of extremely low density (minimum of 0.12 mg cm −3 ), super recyclable compressibility and multifunctionality of combining the thermal insulation, sound absorption, emulsion separation and elasticity-responsive electric conduction, all originating from the synergistic effect of hierarchical cellular fibrous networks and well-bonded nanofibres. Formation of hierarchical cellular-structured FIBER NFAs We designed the FIBER NFAs based on three criteria: (1) the nanofibres must assemble into a 3D aerogel with an open-cell cellular architecture, (2) the nanofibres in the aerogels must be isotropically bonded with each other to form elastic interconnected networks rather than simply stack together and (3) the cellular architecture of the aerogels must not collapse during any post-treatment processing. The first requirement was satisfied by a versatile, readily accessible and gelation-free fibrous freeze-shaping method, which involved the homogenization of nanofibres, the freeze-drying assembly and the final in situ crosslinking. To satisfy the other two criteria—the formation of stable bonded elastic fibrous networks—we combined the unique properties of organic nanofibres (elastic and easy to bond together) with those of inorganic nanofibres (stiff and thermally stable) to yield hybrid fibrous networks with robust elasticity and stability. 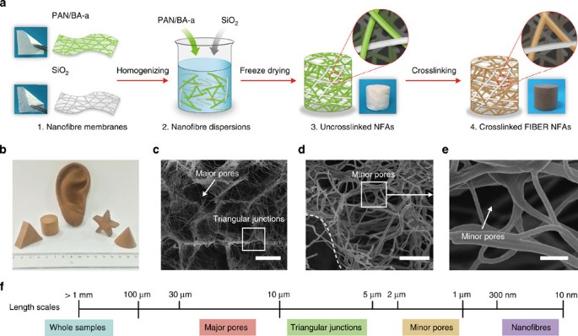Figure 1: Design, processing and cellular architectures of FIBER NFAs (ρ=9.6 mg cm−3). (a) Schematic showing the synthetic steps. (1) Flexible PAN/BA-a and SiO2nanofibre membranes are produced by electrospinning. (2) Homogeneous nanofibre dispersions are fabricated via high-speed homogenization. (3) Uncrosslinked NFAs are prepared by freeze drying nanofibre dispersions. (4) The resultant FIBER NFAs are prepared by the crosslinking treatment. (b) An optical photograph of FIBER NFAs with diverse shapes. (c–e) Microscopic architecture of FIBER NFAs at various magnifications, showing the hierarchical cellular fibrous structure. (f) Schematic representation of the dimensions of relevant structures. Scale bars, 20 μm (c), 5 μm (d) and 1 μm (e). Figure 1a describes the synthesis pathway. Polyacrylonitrile (PAN) nanofibres were selected as the major precursors to construct the elastic fibrous networks, and the bifunctional benzoxazine (BA-a) was blended into PAN nanofibres as a novel in situ crosslinking agent. Rigid SiO 2 nanofibres were introduced into aerogels to enhance their structural stability. The as-prepared PAN/BA-a and SiO 2 electrospun nanofibre membranes were first homogenized in a water/ tert -butanol mixture to form well-dispersed nanofibre despersions and then freeze dried into an uncrosslinked NFA. (see details in Supplementary Figs 1–3 and in Supplementary Methods ). On freezing, the nanofibres in the dispersions were rejected from the moving solidification front and accumulated between the growing cellular solvent crystals, which was governed by complex and dynamic liquid-fibre and fibre–fibre interactions [7] , [27] . By carefully controlling both the dispersity of the nanofibres and the freezing conditions, the NFAs with good formability were readily obtained (see Supplementary Fig. 4 and Supplementary Methods ). Figure 1: Design, processing and cellular architectures of FIBER NFAs ( ρ =9.6 mg cm −3 ). ( a ) Schematic showing the synthetic steps. (1) Flexible PAN/BA-a and SiO 2 nanofibre membranes are produced by electrospinning. (2) Homogeneous nanofibre dispersions are fabricated via high-speed homogenization. (3) Uncrosslinked NFAs are prepared by freeze drying nanofibre dispersions. (4) The resultant FIBER NFAs are prepared by the crosslinking treatment. ( b ) An optical photograph of FIBER NFAs with diverse shapes. ( c – e ) Microscopic architecture of FIBER NFAs at various magnifications, showing the hierarchical cellular fibrous structure. ( f ) Schematic representation of the dimensions of relevant structures. Scale bars, 20 μm ( c ), 5 μm ( d ) and 1 μm ( e ). Full size image To bring about further physical bonding among the fibres, the obtained uncrosslinked NFAs were heated at 240 °C for 1 h to form crosslinked 3D fibrous networks, endowing the resultant FIBER NFAs with elastic resilience ( Supplementary Fig. 5 ). Two synchronous conversions occurred during this process: the preoxidation of PAN and the polymerization of BA-a. As a result of the heat treatment in air, the thermoplastic PAN fibres were converted into thermosetting ladder-structured fibres via cyclization [28] . In addition, the in situ polymerization of the BA-a monomers in the PAN fibres led to the formation of Mannich bridged polybenzoxazine (PBZ) and finally cemented the adjacent nanofibres [29] , [30] . Evidence of the formation of cyclized PAN and PBZ also arose from Fourier transform infrared spectra and differential scanning calorimetry analyses (see Supplementary Fig. 6 and Supplementary Discussions ). Significantly, the PAN nanofibres tended to generate dramatic heat shrinkage in the axial direction, whereas the thermally stable SiO 2 nanofibres acted as a rigid support to prevent the fibrous networks from collapsing ( Supplementary Fig. 7 ). We observed that adding 25 wt% SiO 2 fibres to the aerogel could guarantee stable FIBER NFAs. Due to the simplicity of the assembly process in our methodology and the facile availability of electrospun nanofibres, great versatility in controlling the shapes and scaling up the synthesis of aerogels was possible. As illustrated in Fig. 1b , integrated FIBER NFAs with desired shapes, such as pentagonal prisms, cones, cubes, triangular prisms and intricate ear-like shapes, were readily prepared. More significantly, FIBER NFAs can be easily scaled up by simply using a large shaping mould. For example, we prepared a large FIBER NFA with a volume of 2,000 cm 3 using a mould of a 2-L plate ( Supplementary Fig. 8 ). It is noteworthy that fibrous freeze shaping also simultaneously induces the nanofibres to be organized in a unique cellular architecture on both the nano and micro scales. Figure 1c–e presents typical scanning electron microscope (SEM) images of the FIBER NFAs with a density of 9.6 mg cm −3 . The cellular architecture exhibited an obvious open-cell geometry with a major cellular pore size of 10–30 μm, and these cells were highly interconnected with each other through triangular junctions ( Fig. 1c and Supplementary Fig. 9 ). Zooming in on a single triangular junction revealed that the junction consisted of numerous minor cellular pores with sizes of 1–2 μm ( Fig. 1d,e ). The significant difference between FIBER NFAs and other cellular aerogels is the unique fibrous cell walls that consist of similar minor cellular pores, despite the thickness of the cell wall being ~10 times thinner than that of traditional polymeric foams (10–50 μm) (refs 31 , 32 ) ( Supplementary Fig. 10 ). Figure 1f also contains scale bars showing all the relevant sizes within these hierarchical cellular structures. In conjunction with the anisotropic structure of nanofibres, the principle of the fibrous freeze-shaping process that has previously been proposed for other nanoparticle dispersions can be extended to elucidate the formation of this unique cellular structure [7] , [27] , [33] . A simple model of formation mechanism of the hierarchical cellular structure from nanofibre dispersions is schematically presented in Supplementary Fig. 11 . Characterization of superelasticity We hypothesize that the robust hierarchical cellular structure is responsible for the outstanding mechanical properties of the FIBER NFAs, a structure that allows for large deformations without fractures. In dramatic contrast to the brittle nature of traditional colloidal aerogels, the FIBER NFAs can bear a compressive strain ( ε ) as high as 80% and can recover their original volume after the release of the stress ( σ ), as shown in insets of Fig. 2a and Supplementary Movie 1 . 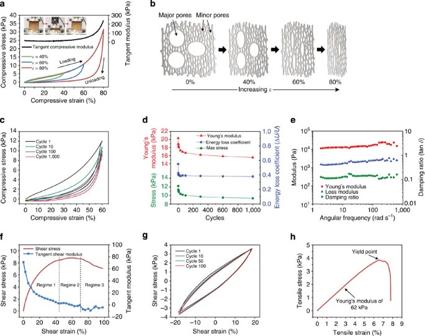Figure 2: Compressive, shear and tensile mechanical properties of the FIBER NFAs (ρ=9.6 mg cm−3). (a) Compressiveσand dσ/dεversusεcurves for the FIBER NFAs. Insets: photographs of the FIBER NFAs under a compressing and releasing cycle (ε=80%). (b) Schematic description of the changes in the hierarchical cellular structure with compressive deformation. (c) 1,000 cyclic compressive fatigue test withεof 60%. (d) History of the Young’s modulus, maximum stress and energy loss coefficient as a function of the compressive test cycles. (e) Dynamic rheological compressive behaviours with oscillatoryεof ±3%. (f) Shearσand dσ/dεversusεcurves for the FIBER NFAs. (g) 100 cyclic shear fatigue test with oscillatoryεof ±20%. (h) Tensileσ–εcurve for the FIBER NFAs. Figure 2a presents plots of the compressive σ–ε curves for the FIBER NFAs at set ε maxima of 40, 60 and 80%, revealing two characteristic deformation regimes typically observed in open-cell foams [10] , [34] : a Hookean or linear elastic regime for ε <60% with a stable tangent modulus (d σ/ d ε ) of ~30 kPa and a densification regime for ε >60% with σ and the d σ/ d ε increasing steeply. The maximum σ was 10.6 kPa for the first elastic regime and 36.1 kPa at 80% strain; these values were significantly higher than those of other fibrous aerogels with similar densities [11] , [35] . Figure 2: Compressive, shear and tensile mechanical properties of the FIBER NFAs ( ρ =9.6 mg cm −3 ). ( a ) Compressive σ and d σ /d ε versus ε curves for the FIBER NFAs. Insets: photographs of the FIBER NFAs under a compressing and releasing cycle ( ε =80%). ( b ) Schematic description of the changes in the hierarchical cellular structure with compressive deformation. ( c ) 1,000 cyclic compressive fatigue test with ε of 60%. ( d ) History of the Young’s modulus, maximum stress and energy loss coefficient as a function of the compressive test cycles. ( e ) Dynamic rheological compressive behaviours with oscillatory ε of ±3%. ( f ) Shear σ and d σ/ d ε versus ε curves for the FIBER NFAs. ( g ) 100 cyclic shear fatigue test with oscillatory ε of ±20%. ( h ) Tensile σ–ε curve for the FIBER NFAs. Full size image To provide insight into the mechanism of elasticity, we performed in situ SEM observations under increasing compressive ε up to 80% ( Supplementary Figs 12 and 13 ). We also quantified the strain-induced structural reorganization using the two-dimensional small angle X-ray scattering (SAXS) measurements (see details in Supplementary Figs 14 and 15 and Supplementary Discussions ). The circular SAXS pattern for the FIBER NFAs without strain ( ε =0%) indicated an isotropic orientation structure [36] . Subsequently, the compression restricted the fibres to orient increasingly in a plane perpendicular to the compressive direction. Up to ε =60%, the open-cell geometric, interconnected major cellular pores were gradually compacted and deformed ( Supplementary Fig. 13a ); correspondingly, asymmetric SAXS patterns were observed [37] , [38] . Beyond 60% ε , the major pores were densely packed and almost parallel to one another, thus inducing the compaction of the minor pores in the triangular junctions ( Supplementary Fig. 13b ). The densification of the cellular structure at ε= 80% led to an abrupt SAXS intensity increase and obviously elliptical patterns, showing the enhancement in the structural orientation [38] , [39] . Moreover, the SAXS intensities exhibited identical variations under a compressing and releasing cycle, further demonstrating the remarkable structural resilience of the FIBER NFAs. These SEM observations and SAXS features up to 80% strain corresponded well with the two-regime σ–ε curve. From these results, we propose that the strain is absorbed at a high level by the deformation of major cellular pores and beyond 60% strain by the densification of minor pores ( Fig. 2b ). The FIBER NFAs were subjected to a cyclic compression test with 1,000 loading–unloading fatigue cycles at a large ε of 60% with a loading rate of 300 mm min −1 ( Fig. 2c ), and they exhibited slight plastic deformation (4.8% at 100th, 14.5% at 1,000th), highlighting their structural robustness. In comparison, a plastic deformation of 20–30% at ε ≈60% is typical for polymeric foams [10] , and other fibrous foams exhibit plastic deformation of larger than 20% at similar strains [11] . Similarly, no significant decrease in the stiffness or strength was observed for FIBER NFAs by 1,000 cyclic compressions; they retained over 75% of the original Young’s modulus and maximum stress ( Fig. 2d ). The FIBER NFAs also exhibited obvious hysteresis during the compression experiments. For the first cycle, we estimated the work performed in the compression to be 2.71 mJ cm −3 and the energy dissipation to be 1.49 mJ cm −3 , yielding an energy loss coefficient (Δ U / U ) of 0.55. This large energy dissipation resulted from the viscoelasticity of the organic nanofibrous networks. After 10 cycles, a nearly constant energy loss coefficient of ~0.4 was calculated, which was higher than that for typical carbon or metal foams [16] , [40] . Further dynamic compressive viscoelastic measurements revealed that the Young’s modulus ( E′ ) and loss modulus ( E″ ) were nearly stable and were independent of the angular frequency ( ω ) over the three decades of accessible ω from 1.8 to 628 rad s −1 ( Fig. 2e ), and E′ was one order of magnitude higher than E″ . A damping ratio of 0.1–0.15 over the entire tested range of angular frequencies implied that the elastic response was predominant and that the FIBER NFAs contained strong, viscoelastic networks. Moreover, the dynamic tests also revealed that the FIBER NFAs recovered their original shape at least at the speed of the compression head, which ranged from 4.32 mm min −1 ( ω =1.8 rad s −1 ) to 1,440 mm min −1 ( ω =628 rad s −1 ). These prominent recovery rates were significantly higher than those of conventional polymeric foams [10] (<100 mm min −1 ) and carbon aerogels [11] , [34] (<700 mm min −1 ). In addition, the FIBER NFAs underwent a transverse contraction when compressed in one direction and exhibited a negative Poisson’s ratio ( Supplementary Fig. 16 ), which has also been observed in other cellular foams due to the inverting of the cell walls [10] , [41] . We performed shear and tensile measurements ( Supplementary Fig. 17 ) to further characterize the structure and properties of the FIBER NFAs. As observed in Fig. 2f , the shear σ–ε curve exhibited three typical regimes as the ε was increased [42] , [43] : an elastic deformation stage at ε <40%, a plastic plateau near the yield point with ε of 40–70%, and the last fracture stage with a rapid decrease of σ . The d σ/ d ε curve exhibited three distinct regimes with positive, zero and negative values, further confirming the three-stage shear deformation. The maximum shear σ of the FIBER NFAs was 8.82 kPa with a large yield shear ε of 61%. Moreover, the cyclic shear test with an oscillatory ε of ±20% exhibited identical σ–ε behaviour even after 100 cycles, which demonstrated the excellent fatigue resistance to shear deformation ( Fig. 2g ). These oscillatory shear σ–ε curves showed nonlinearity and closed hysteresis without abrupt changes, which are typical of viscoelastic, energy-dissipative and highly deformable materials, such as rubber [43] . The tensile σ–ε curve presented in Fig. 2h exhibited that, as the ε increased, the σ first increased linearly with a robust Young’s modulus of 62 kPa, and fracture occurred immediately after the σ reached its maximum yield value of 4.33 kPa. In addition, the fracture behaviour in tension was quite different from that in compression/shear. The tensile stress caused a fast and brittle fracture, whereas the compression/shear stress led to a progressive crushing. This difference in fracture behaviours is typically observed in other cellular foams and is attributed to the diverse mechanisms of yielding and fracturing [10] , [42] , as demonstrated in Supplementary Discussions . Tunable densities of FIBER NFAs The unique advantages of the mechanically robust, hierarchical cellular structure can be further demonstrated by the successful synthesis of FIBER NFAs at ultra-low densities with no requirement for any additional binders. We prepared FIBER NFAs with various densities (0.53–9.6 mg cm −3 ) simply by adjusting the concentrations of the starting nanofibre dispersions, and their mechanical properties are summarized in Supplementary Fig. 18 and Supplementary Table 1 . Plotting the relative compressive modulus ( E / E s ) of various fabricated FIBER NFAs versus their relative density ( ρ / ρ s ) revealed that the modulus scaled as E / E s ~( ρ / ρ s ) [2] ( Fig. 3a ), indicating a cellular-dominated mechanical behaviour similar to that of open-cell cellular foams [10] , [44] . This scaling law also affects the structural stability of self-supporting cellular materials, imposing a lower bound on density [7] , [9] . In contrast, most existing ultralight materials [45] , [46] , [47] , such as carbon foams and silica aerogels, follow a steeper scaling of E / E s ~( ρ / ρ s ) [3] ( Fig. 3a ) due to the inefficient load transfer between ligaments. Moreover, thanks to the scalable synthesis methodology, the E / E s ~( ρ / ρ s ) [2] scaling law was further vertically regulated on the E ~ ρ map. For example, we fabricated a series of softer FIBER NFAs using a flexible alkyl benzoxazine (BA-oda) as the crosslinking agent, which exhibited good E / E s ~( ρ / ρ s ) [2] scaling with a lower modulus. In addition, we believe that further tuning of the intrinsic properties of nanofibres by changing the fibre materials and crosslinking agents could yield varieties of FIBER NFAs with a wide range of designed mechanical properties. 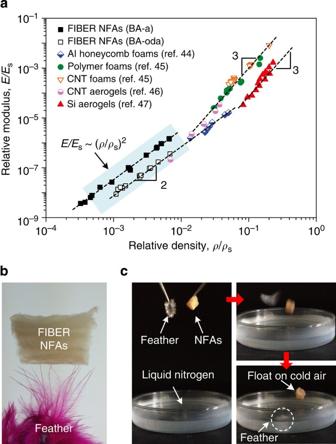Figure 3: Mechanical properties of FIBER NFAs with various densities. (a) The relative modulus (defined as the measured Young’s modulus,E, divided by the Young’s modulus of the constituent solid,Es) of selected cellular materials at low relative densities. (b) A 20-cm3FIBER NFA (ρ=0.12 mg cm−3) stands on the tip of dyed feathers. (c) Photographs demonstrate that the ultralight FIBER NFAs (ρ=0.12 mg cm−3) can even float on cold air. Figure 3: Mechanical properties of FIBER NFAs with various densities. ( a ) The relative modulus (defined as the measured Young’s modulus, E , divided by the Young’s modulus of the constituent solid, E s ) of selected cellular materials at low relative densities. ( b ) A 20-cm 3 FIBER NFA ( ρ =0.12 mg cm −3 ) stands on the tip of dyed feathers. ( c ) Photographs demonstrate that the ultralight FIBER NFAs ( ρ =0.12 mg cm −3 ) can even float on cold air. Full size image Following the accessibility of ultralight aerogels with densities below 10 mg cm −3 , the next goal is to achieve ultra-flyweight aerogels with a density less than 0.5 mg cm −3 . The lowest density of FIBER NFAs we have obtained is 0.12 mg cm −3 ( Fig. 3b , Supplementary Fig. 19 and Supplementary Movie 2 ), corresponding to a porosity of 99.992%, which is obviously lower than that of previously reported ultralight aerogels [6] , [8] . In addition, the ultralight feature was further confirmed using a designed concept experiment, as illustrated in Fig. 3c . Compared with light feathers, the FIBER NFAs with a density of 0.12 mg cm −3 can easily float on cold air and behave as a boat, relying only on the minute density difference between the room and cold air (see Supplementary Movies 3 and 4 ). Significantly, the efficient heat insulation also contributed to the floating demonstration because the air trapped in the aerogels was difficult to cool down and provided stable buoyancy. Multifunctionality of FIBER NFAs Aerogels are among the most well-known thermal insulation materials with extraordinarily low thermal conductivity originating from their high porosity [3] , [48] . As illustrated in Fig. 4a , the FIBER NFAs with a density of 0.12 mg cm −3 exhibited a prominent thermal conductivity of 0.026 W m −1 K −1 , which is similar to that of air at ambient conditions (0.023 W m −1 K −1 ). We attributed this result to the extremely high porosity of the FIBER NFAs (99.992%). When the density of the FIBER NFAs was increased to 9.6 mg cm −3 , the thermal conductivity slightly increased to 0.0304 W m −1 K −1 because of the decrease of the porosity (99.36%). Benefiting from the ultralight feature of the FIBER NFAs, the thermal insulation performance per unit mass of the FIBER NFAs (0.12 mg cm −3 ) was estimated to be one or two orders of magnitude greater than that of commonly used insulation materials [10] , [48] ( Supplementary Table 2 ), suggesting their use as promising lightweight thermal insulation materials in a wide range of applications. 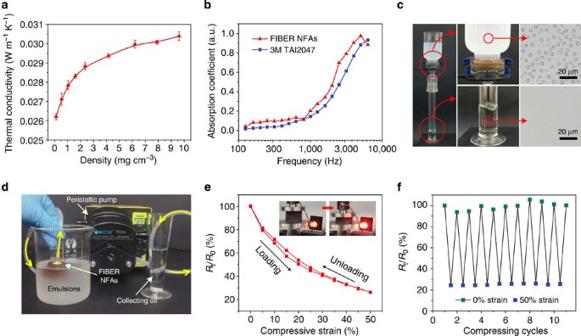Figure 4: Multifunctionality of combining the thermal insulation, sound absorption, emulsion separation and electric conduction. (a) The thermal conductivities of the FIBER NFAs in air as a function of density. (b) Frequency dependence of the sound absorption coefficient of the FIBER NFAs (ρ=9.6 mg cm−3) and commercial 3M TAI2047 non-wovens. (c) Separation apparatus with the facile gravity-driven separation of water-in-oil emulsions using the FIBER NFAs (ρ=9.6 mg cm−3). (d) Photograph of the oil collection apparatus continuously collecting pure oil from water-in-oil emulsions. (e)Rt/R0hysteresis of the CNFAs (ρ=5.1 mg cm−3) as a function of strain under a compressing and releasing cycle (ε=50%). The insets show that the brightness increases on compression of the CNFAs. (f)Rt/R0of the CNFAs when repeatedly compressed (ε=50%) over 10 cycles. Figure 4: Multifunctionality of combining the thermal insulation, sound absorption, emulsion separation and electric conduction. ( a ) The thermal conductivities of the FIBER NFAs in air as a function of density. ( b ) Frequency dependence of the sound absorption coefficient of the FIBER NFAs ( ρ =9.6 mg cm −3 ) and commercial 3M TAI2047 non-wovens. ( c ) Separation apparatus with the facile gravity-driven separation of water-in-oil emulsions using the FIBER NFAs ( ρ =9.6 mg cm −3 ). ( d ) Photograph of the oil collection apparatus continuously collecting pure oil from water-in-oil emulsions. ( e ) R t / R 0 hysteresis of the CNFAs ( ρ =5.1 mg cm −3 ) as a function of strain under a compressing and releasing cycle ( ε =50%). The insets show that the brightness increases on compression of the CNFAs. ( f ) R t / R 0 of the CNFAs when repeatedly compressed ( ε =50%) over 10 cycles. Full size image Sound absorption or dissipation is one of the key functions of cellular foams, especially for materials containing open-cell porous channels [40] , [49] . The current sound absorption materials are mainly meltblown non-wovens, and 3M Thinsulate TAI2047 felts [50] are well-known lightweight materials that have a thickness of 10 mm and an areal density of 210 g m −2 . Strikingly, the FIBER NFAs with half of the thickness (5 mm) and a quarter of the areal density (48 g m −2 ) exhibited a clearly higher sound absorption coefficient than TAI2047 over the entire testing frequency (100–6,300 Hz; Fig. 4b and Supplementary Fig. 20 ). This result was attributed to the hierarchical cellular fibrous networks that were composed of numerous connected resonant microchannels. Acoustic waves enter through these channels and are converted into heat by viscous and thermal losses as they move through the aerogels; ultimately, they are efficiently dissipated [49] , [51] . We thus envisage their use for sound absorption in special weight-concerned fields such as the aviation and aerospace industries. Another unique feature of the FIBER NFAs was their robust selective wettability. Because of the low surface energy of the PBZ [52] , the FIBER NFAs exhibited hydrophobicity, with a water contact angle of 145°, and superoleophilicity, with an oil contact angle of 0° ( Supplementary Fig. 21a ). Thus, these materials exhibited low adhesion to a water droplet with no permeation, whereas an oil droplet rapidly permeated into the sample within 9 ms ( Supplementary Fig. 21b and Supplementary Movie 5 ). Moreover, the hierarchical cellular structure provided numerous microporous channels for the liquid transportation; thus, effective separation of oil/water emulsions by the FIBER NFAs was expected. Figure 4c showed the solely gravity-driven separation of surfactant-stabilized water-in-oil emulsions (petroleum ether was used as an example) using the FIBER NFAs; the oil immediately permeated through the aerogels, whereas the emulsified water droplets were retained above ( Supplementary Movie 6 ). The FIBER NFAs exhibited a high separation flux of 8,100±160 l m −2 per hour, which was obviously higher than that of other pressure-driven separation materials [53] , [54] ( Supplementary Fig. 22 ). Furthermore, the mechanically robust FIBER NFAs achieved the collection of pure oil from the oil/water emulsions via a novel, continuous and convenient pumping method ( Fig. 4d and Supplementary Movie 7 ), thus implying their potential usefulness for treating real emulsified oil/water mixtures on a mass scale, particularly in environmental protection and pollution control applications [54] , [55] . We further demonstrate that the as-prepared FIBER NFAs can be facilely carbonized to yield conductive carbon NFAs (CNFAs) because the PAN is a well-known precursor to prepare graphitized carbon fibres [28] , [56] . After pyrolysis at 850 °C, the resultant CNFAs still retained the unique hierarchical cellular structure ( Supplementary Fig. 23 ); thus, the robust elasticity was well inherited. Note that the prominent structural stability of aerogels during carbonization is derived from the sturdy SiO 2 nanofibres, which remain stable under extreme conditions. Significantly, the carbonization brings the elasticity-dependent electrical conductivity of CNFAs, which exhibited a promising initial conductivity of 0.25 S cm −1 . The normalized electrical resistance ( R t / R 0 ) decreased dramatically (70%) with an increase in strain to 50% and recovered well during the unloading process ( Fig. 4e ). This was because the compression created numerous new temporary contacts among fibres, and added to the previously existing conduction paths throughout the sample, finally decreased the electrical resistance. A light-emitting diode was illumined using a 3-V circuit when connected with the CNFAs, and its brightness fluctuated as the aerogels were compressed and released (insets in Fig. 4e and Supplementary Movie 8 ). In addition, the response of R t / R 0 for the CNFAs was also quite constant over multiple cycles of compression ( Fig. 4f ), demonstrating the promising structural stability. These results support the use of CNFAs as ultralight, flexible pressure-responsive sensors for various applications. The successful synthesis of FIBER NFAs provides a versatile platform for exploring the applications of nanofibres in a self-supporting, structurally adaptive and 3D macroscopic form. In this work, PAN/SiO 2 -based FIBER NFAs were developed as a model system for proof-of-concept; in considering the ease of scalable synthesis of electrospun nanofibres from various materials, our discovery will thus pave the way for new types of nanofibre-based functional aerogels for use in various applications. For instance, biocompatible nanofibre membranes (such as poly(lactic acid) and polycaprolactone) have been widely used as tissue engineering scaffolds; thus, creating 3D FIBER NFAs using these biocompatible nanofibres could provide a better mimic of the extracellular matrix by offering another direction for cell interactions, migration, and morphogenesis [25] , [26] . Moreover, similar to the synthesis of CNFAs, a variety of inorganic NFAs can be also expected by the calcination of relevant precursor FIBER NFAs. Furthermore, other functional materials (for example, Au, TiO 2 and Fe 3 O 4 nanoparticles) can be readily incorporated into the open-cell void space, offering plenty of room to fabricate many novel fibre-particle composite FIBER NFAs. In conclusion, we have demonstrated a gelation-free, synergistic assembly strategy for the scalable fabrication of superelastic, hierarchical cellular-structured FIBER NFAs through the combination of electrospun nanofibres and the fibrous freeze-shaping method. For the first time, the intrinsically lamellar deposited electrospun nanofibres are reconstructed into 3D fibrous bulk aerogels with tunable densities and desirable shapes on a large scale. With their ultra-low density, super recyclable compressibility and unique multifunctionality in terms of the combination of thermal insulation, sound absorption, emulsion separation and elasticity-responsive electric conduction, we envision that such exceptional FIBER NFAs will open up numerous opportunities for a range of applications in dampers, electrodes, heat insulators, sieves, absorbents, separators, tissue engineering scaffolds and pressure sensors. Preparation of PAN/BA and SiO 2 nanofibres BA-a and BA-oda monomers were synthesized using bisphenol-A, amine and paraformaldehyde via the Mannich reaction, see details in Supplementary Methods . For PAN/BA-a composite nanofibres, the precursor solution was prepared by dissolving PAN ( M n =90,000, Spectrum) and BA-a in dimethylformamide at concentrations of 6 and 1.5 wt%, respectively. The electrospinning was performed using a DXES-3 spinning machine (SOF Nanotechnology Co., China). The solution was loaded into a syringe capped with a 6-G metal needle with a controllable feed rate of 2 ml per hour. A high voltage of 25 kV was applied to the needle tip, resulting in the generation of a continuous jetting stream. The resultant nanofibres were deposited onto the aluminium foil-covered grounded metallic rotating roller with a rotation rate of 50 r.p.m. at a 15-cm spinneret-collector distance. The relevant temperature and humidity during electrospinning were 25±2 °C and 45±2%, respectively. Similarly, the PAN/BA-oda composite nanofibres were prepared using the same process. In the case of SiO 2 nanofibres, the precursor solution was prepared by dissolving polyvinyl alcohol (PVA, M n =86,000, Wako) in pure water at 80 °C with vigorous stirring. A silica precursor solution with a molar composition of tetraethyl orthosilicate (TEOS):H 3 PO 4 :H 2 O=1:0.01:11 was prepared via hydrolysis and polycondensation by dropwise addition of H 3 PO 4 to TEOS with stirring at room temperature for 12 h. The resultant silica precursor solution was added to the PVA solution (weight ratio of 1:1) and stirred for another 4 h. The electrospinning was subsequently performed under an applied voltage of 17 kV and at a controllable feed rate of 1 ml per hour. The resultant hybrid nanofibres were deposited onto the aluminium foil-covered grounded metallic rotating roller with a rotation rate of 50 r.p.m. at a 20-cm spinneret-collector distance. The relevant temperature and humidity during electrospinning were 25±2 °C and 45±2%, respectively. To obtain pure SiO 2 nanofibres, the as-spun nanofibres were calcined at 800 °C in air by gradually increasing the temperature at a heating rate of 5 °C min −1 to remove the PVA. Fabrication of FIBER NFAs by fibrous freeze-shaping method The detailed fabrication process is described in Supplementary Figs 1–4 and Supplementary Methods . In a typical experiment for the synthesis of FIBER NFAs (BA-a as crosslinking agent) with a density of 9.6 mg cm −3 , 0.75 g of PAN/BA-a and 0.25 g of SiO 2 nanofibre membranes were cut into 1 × 1 cm 2 pieces, and were dispersed in 100 ml of a water/ tert -butanol mixture (weight ratio of 4:1) by homogenizing the mixture for 20 min at 13,000 r.p.m. using an IKA T25 homogenizer, yielding uniform nanofibre dispersions. Next the dispersions were poured into the desired mould, frozen in liquid nitrogen, annealed at –25 °C for 1 h and then freeze dried (Labconco FreeZone freeze-drying system) for 48 h to obtain the uncrosslinked NFAs. Finally, they were heated at 240 °C for 1 h in air, giving rise to the crosslinked FIBER NFAs. Other FIBER NFA samples with densities ranging from 0.12 to 9.6 mg cm −3 were fabricated by adjusting the concentrations of the original nanofibre dispersions. To obtain the CNFAs, the as-prepared FIBER NFAs were calcined at 850 °C for 30 min at a heating rate of 2 °C min −1 under Ar flow (0.002 m 3 min −1 ). Characterization The compression tests were performed using Instron 3365 testing system equipped with two flat-surface compression stages and 100-N load cells. Cylindrical FIBER NFA samples with diameters of ~28 mm were used. The σ – ε curves with ε =40, 60 and 80% were measured at a strain rate of 30 mm min −1 and a 3% prestrain was applied to make a uniform flat contact between the compression heads and the sample and to prevent slipping of the sample. A 1,000-cycle loading–unloading fatigue cyclic test was performed by measuring σ versus ε =60% at a strain rate of 300 mm min −1 with a 3% prestrain. Dynamic compressive viscoelastic measurements of the FIBER NFAs were performed using a TA-Q800 DMA instrument with a parallel-plate compression clamp; the gap distance between the two plates was fixed at 4 mm. E′ and E″ as a function of ω from 1.8 to 628 rad s −1 were measured with an oscillatory strain of ±3% and a prestrain of 5%. The shear mechanical properties were measured using a TA-Q800 DMA instrument with a sandwich shear clamp; the thickness of the test sample was 4 mm, as shown in Supplementary Fig. 17a . The shear σ – ε curve was measured at a maximum ε of 100% with a ε rate of 50% min −1 . A 100-cycle fatigue shear test was performed with an oscillatory shear ε of ±20% at a strain rate of 200% min −1 ; the initial ε of the fatigue test was set to 20%. The tensile test was performed on an Instron 3365 testing system according to the ISO 1798:2008 standard, as illustrated in Supplementary Fig. 17b . Rectangular samples with thicknesses of 10 mm were used, and the tensile loading rate was 1 mm min −1 . The weights of the FIBER NFAs were determined using a Mettler Toledo Micro balance (AT-20) with a readability of 2 μg. The density (apparent density) of the FIBER NFAs was measured on the basis of the ISO 845:2006 standard, which was calculated by the weight of solid contents without including the weight of air entrapped in pores. As the samples were weighted in air, the weight of air was automatically eliminated. Note that this standard is suit for cellular materials, such as polymer foam and aerogels, and the comparison of apparent density to absolute density that is typically for bulk materials is inappropriate. The porosity and compression work of FIBER NFAs was determined based on the standard practice for cellular materials, as demonstrated in the Supplementary Methods . The SEM images were examined using a Hitachi S4800 field-emission SEM system. Fourier transform infrared spectra were collected with a Nicolet 8700 spectrometer in the range 4,000–400 cm −1 . Differential scanning calorimetry measurements were performed with a TA-Q200 differential scanning calorimeter. The two-dimensional SAXS measurements were performed at the BL16B1 beamline in the Shanghai Synchrotron Radiation Facility; the experimental details presented in Supplementary Figs 14 and 15 and in Supplementary Discussions . The heat insulation coefficient was determined on a Hot Disk TPS2500S using the transient plane source method. The sound absorption coefficients were measured using the impedance tube technique (SW260, BSWA) and the transfer function method. Measurements of the water contact angle (3 μl) and oil contact angle (3 μl, petroleum ether) were performed using a Kino SL200B contact angle goniometer. The details for emulsion separation experiments were presented in the Supplementary Methods . The elasticity-dependent electrical conductivity was determined using a two-probe method. We attached copper wire leads to the flat surfaces of the cylindrical CNFAs with silver paste, and these CNFAs were loaded between the two compression heads of Instron 3365 system with a prestrain of 3%. The EC-Lab software and a Fluke ohmmeter were used to measure the resistance of the aerogels as a function of ε . How to cite this article: Si, Y. et al . Ultralight nanofibre-assembled cellular aerogels with superelasticity and multifunctionality. Nat. Commun. 5:5802 doi: 10.1038/ncomms6802 (2014).